Reconstitution of a 10-gene pathway for synthesis of the plant alkaloid dihydrosanguinarine inSaccharomyces cerevisiae Benzylisoquinoline alkaloids (BIAs) represent a large class of plant secondary metabolites, including pharmaceuticals such as morphine, codeine and their derivatives. Large-scale production of BIA-based pharmaceuticals is limited to extraction and derivatization of alkaloids that accumulate in planta . Synthesis of BIAs in microbial hosts could bypass such limitations and transform both industrial production of BIAs with recognized value and research into uncharacterized BIAs. Here we reconstitute a 10-gene plant pathway in Saccharomyces cerevisiae that allows for the production of dihydrosanguinarine and its oxidized derivative sanguinarine from ( R,S )-norlaudanosoline. Synthesis of dihydrosanguinarine also yields the side-products N -methylscoulerine and N -methylcheilanthifoline, the latter of which has not been detected in plants. This work represents the longest reconstituted alkaloid pathway ever assembled in yeast and demonstrates the feasibility of the production of high-value alkaloids in microbial systems. Many pharmaceutical drugs are isolated directly from plants or are semisynthetic derivatives of natural products [1] , [2] . Information from New Drug Applications and clinical trials is evidence that the pharmaceutical industry continues to use natural products as a source of new drug leads [3] . However, the pipeline of drug discovery is difficult to sustain, due to technical challenges in isolating new compounds with diverse structures and complex chemistries in sufficient quantities for screening [4] . Next generation DNA sequencing technology has provided rapid access to the genetic diversity underpinning the immense biosynthetic capacity of plants and microbes [5] , [6] . Although Saccharomyces cerevisiae has traditionally been used for the biosynthesis of simple molecules derived from central metabolism [7] , advances in recombinant DNA technology streamlining the cloning of large DNA sequences make this microbe an attractive platform for functional characterization of enzymes as well as the reconstitution of complex metabolic pathways [8] , [9] . When combined with genetic information on an ever-increasing number of species, microbial hosts provide new opportunities for the discovery and production of diverse and complex natural products. A recent example demonstrating the power of these combined technologies is the high-level production of the artemisinin antimalarial drug precursor artemisinic acid in yeast [10] . Benzylisoquinoline alkaloids (BIAs) are a diverse class of plant secondary metabolites including such pharmaceuticals as the antitussive codeine, the analgesic morphine, the antitussive and anticancer drug noscapine [11] and the antibacterial and potential antineoplastic drugs berberine and sanguinarine [12] . Their complex molecular backbone and the presence of multiple stereocentres makes the complete chemical synthesis of most BIAs commercially unfeasible [13] , [14] , [15] . Consequentially, plant extraction is the only commercial source of BIAs, which limits the diversity of BIA structures available for drug discovery due to their low abundance [16] . The pharmaceutical value of BIAs and advances made in the elucidation of their biosynthesis in plants have made these compounds high-value candidates for production using microbial hosts [17] . Despite their structural diversity, BIAs share many common biosynthetic steps and intermediates. Escherichia coli was recently engineered to produce the key BIA intermediate ( S )-reticuline from glucose or glycerol [18] , [19] and co-cultured with S. cerevisiae expressing heterologous enzymes to synthesize ( S )-magnoflorine and ( S )-scoulerine [20] . While production of the key intermediate ( S )-reticuline from simple carbon sources in E. coli is an undeniable success, S. cerevisiae is a more attractive host for BIA synthesis, due to its superior ability to express the cytochrome P450s common in downstream alkaloid synthesis [21] . Strains of S. cerevisiae were also engineered for the production of the BIA intermediates ( R,S )-reticuline and ( S )-scoulerine, and the protoberberine intermediates ( S )-tetrahydrocolumbamine and ( S )-canadine using the fed substrate ( R,S )-norlaudanosoline [22] . However, gaps in biosynthetic pathways and the complexity of multi-gene co-expression in microbial hosts have prevented the production of a more diverse set of BIAs thus far. Sanguinarine is a BIA with recognized antimicrobial activities and potential as an antineoplastic drug [23] , [24] . The last steps in sanguinarine biosynthesis were recently elucidated, laying the groundwork for complete synthesis of this molecule in a heterologous host [25] , [26] , [27] . Here we combine gene discovery with multi-gene heterologous expression in S. cerevisiae to reconstitute a 10-gene BIA pathway for the biosynthesis of dihydrosanguinarine and sanguinarine from the commercial precursor ( R,S )-norlaudanosoline. We also demonstrate the activity of tetrahydroprotoberberine cis - N -methyltransferase (TNMT) towards scoulerine and cheilanthifoline and synthesize N -methylscoulerine and N -methylcheilanthifoline in yeast. The reconstitution of a complex pathway for BIA synthesis in S. cerevisiae represents an important advance towards the production of a broader class of alkaloids in a microbial host. CFS and SPS from opium poppy Sanguinarine biosynthesis from ( S )-scoulerine proceeds with the formation of two methylendioxy bridges catalysed by the P450s cheilanthifoline synthase (CFS) and stylopine synthase (SPS), to yield cheilanthifoline and stylopine, respectively ( Fig. 1 ). Candidate genes encoding opium poppy ( Papaver somniferum ) CFS (PsCFS) and SPS (PsSPS) were isolated from assembled opium poppy root and stem transcriptome databases generated using Illumina GA sequencing. Query amino-acid sequences used to search each database were AmCFS and AmSPS from Argemone mexicana [28] . The selection of candidate genes was guided by the expectation that PsCFS and PsSPS transcripts would occur exclusively or predominantly in opium poppy roots, owing to the lack of sanguinarine accumulation in stems of the plant [29] . A PsCFS candidate corresponding to CYP719A25 shared 84% amino-acid identity with AmCFS and was expressed exclusively in opium poppy roots ( Fig. 2a ). A PsSPS candidate corresponding to CYP719A20 shared 79% amino-acid identity with AmSPS and was expressed predominantly in roots ( Fig. 2a ). 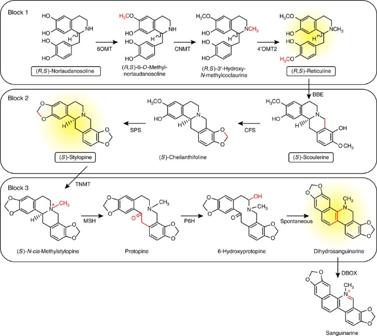Figure 1: Description of the enzyme block strategy used in the reconstitution of the sanguinarine biosynthetic pathway inS. cerevisiae. Enzymes were tested for functional activity by blocks of sequential enzymes and on the basis of availability of feeding substrates. The final product from each block is highlighted. Boxed text indicates alkaloids used as feeding substrates. CFS, cheilanthifoline synthase (CYP710A25); SPS, stylopine synthase (CYP719A20); MSH, (S)-cis-N-methylstylopine 14-hydroxylase (CYP82N4), P6H, protopine 6-hydroxylase (CYP82N2v2); DBOX, dihydrobenzophenanthridine oxidase. P6H is fromE. californica, all other enzymes used in this work are fromP. somniferum. TheP. somniferumcytochrome P450 reductase (CPR) was also expressed for functional expression of cytochromes P450s together with Block 2 and/or 3. Figure 1: Description of the enzyme block strategy used in the reconstitution of the sanguinarine biosynthetic pathway in S. cerevisiae . Enzymes were tested for functional activity by blocks of sequential enzymes and on the basis of availability of feeding substrates. The final product from each block is highlighted. Boxed text indicates alkaloids used as feeding substrates. CFS, cheilanthifoline synthase (CYP710A25); SPS, stylopine synthase (CYP719A20); MSH, ( S )- cis - N -methylstylopine 14-hydroxylase (CYP82N4), P6H, protopine 6-hydroxylase (CYP82N2v2); DBOX, dihydrobenzophenanthridine oxidase. P6H is from E. californica , all other enzymes used in this work are from P. somniferum . The P. somniferum cytochrome P450 reductase (CPR) was also expressed for functional expression of cytochromes P450s together with Block 2 and/or 3. 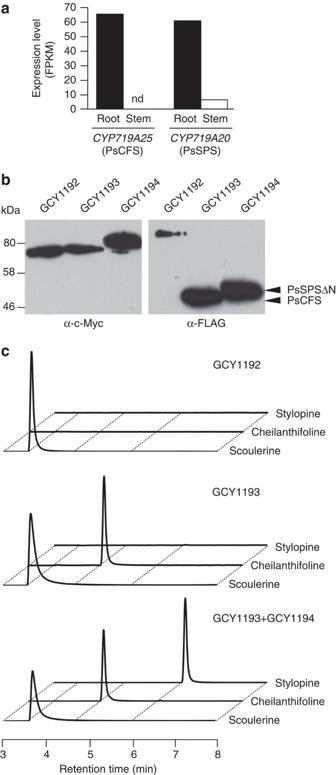Figure 2: Characterization of PsCFS and PsSPS. (a) RNAseq analysis reporting relative transcript abundance of CYP719A25 (PsCFS) and CYP719A20 (PsSPS) in opium poppy roots and stems presented as Fragments Per Kilobase of exons model per Million mapped reads (FPKM). Data presented derive from a single experiment. (b) Immunoblot analysis of microsomal proteins fromS. cerevisiaestrains (i) GCY1192 (expressing PsCPR) (ii) GCY1193 (expressing PsCPR and PsCFS) or (iii) GCY1194 (expressing PsCPR and PsSPSΔN). α-c-Myc and α-FLAG antibodies (1:1,000 dilution) and goat anti-mouse IgG HRP conjugate (1:15,000 dilution) were used to detect CPR, and PsCFS and PsSPS (arrowheads), respectively. Each lane was loaded with ~20 μg of microsomal proteins. (c) LC-MS profiles of enzyme assays of microsomal proteins fromS. cerevisiaestrains (i) GCY1192 (ii) GCY1193 or (iii) a mixture of GCY1193 and GCY1194 incubated with (S)-scoulerine. Abbreviation: nd, not detected. Full size image Figure 2: Characterization of PsCFS and PsSPS. ( a ) RNAseq analysis reporting relative transcript abundance of CYP719A25 (PsCFS) and CYP719A20 (PsSPS) in opium poppy roots and stems presented as Fragments Per Kilobase of exons model per Million mapped reads (FPKM). Data presented derive from a single experiment. ( b ) Immunoblot analysis of microsomal proteins from S. cerevisiae strains (i) GCY1192 (expressing PsCPR) (ii) GCY1193 (expressing PsCPR and PsCFS) or (iii) GCY1194 (expressing PsCPR and PsSPSΔN). α-c-Myc and α-FLAG antibodies (1:1,000 dilution) and goat anti-mouse IgG HRP conjugate (1:15,000 dilution) were used to detect CPR, and PsCFS and PsSPS (arrowheads), respectively. Each lane was loaded with ~20 μg of microsomal proteins. ( c ) LC-MS profiles of enzyme assays of microsomal proteins from S. cerevisiae strains (i) GCY1192 (ii) GCY1193 or (iii) a mixture of GCY1193 and GCY1194 incubated with ( S )-scoulerine. Abbreviation: nd, not detected. Full size image Constructs for the heterologous expression of PsCFS and PsSPS in S. cerevisiae were assembled in a vector harbouring PsCPR ( Table 1 ). Western blot analysis of PsSPS showed that it was poorly expressed. To improve expression, the native N-terminal membrane-spanning domain was swapped with that of lettuce germacrene A oxidase, generating PsSPSΔN. Immunoblot analysis confirmed expression of the recombinant proteins in yeast ( Fig. 2b ). Microsomes were isolated from all three strains and incubated in vitro with ( S )-scoulerine. Scoulerine was converted to cheilanthifoline in the presence of PsCPR and PsCFS, while scoulerine was converted to cheilanthifoline and stylopine in the presence of PsCPR, PsCFS and PsSPS ( Fig. 2c ). No conversion of scoulerine was detected in the negative control. In the present study, PsCFS and PsSPS from opium poppy were used for the reconstitution of dihydrosanguinarine synthesis in S . cerevisiae . Table 1 List of Saccharomyces cerevisiae strains and plasmids used in this study. Full descriptions are available in Supplementary Table 1 Full size table Reconstitution of the dihydrosanguinarine pathway The synthesis of sanguinarine from norlaudanosoline requires 10 enzymatic reactions ( Fig. 1 ). In reconstitution of the pathway, we omitted dihydrobenzophenanthridine oxidase because of its low activity in S. cerevisiae [26] and because dihydrosanguinarine is easily oxidized to sanguinarine ex vivo [30] . We divided the remaining nine reactions into three ‘blocks’ of three sequential enzymes, as illustrated in Fig. 1 . Each block was cloned into a separate plasmid and the cytochrome P450 reductase from P. somniferum (PsCPR) was cloned into a fourth plasmid ( Table 1 ). To confirm functional expression of enzymes, plasmids expressing each of the three blocks were individually transformed into S. cerevisiae and cultures of the strains were supplemented with either ( R,S )-norlaudanosoline, ( S )-reticuline, ( S )-scoulerine or ( S )-stylopine. Functional expression was verified by detection of the expected end products. As negative controls, yeast strains lacking enzyme blocks were incubated with each of the pathway intermediate to evaluate substrate recovery and to assess the relative proportion recovered in cellular extracts versus culture supernatants. Functional expression of individual enzyme blocks Block 1 contains the P. somniferum enzymes 6- O -methyltransferase (6OMT), coclaurine N -methyltransferase (CNMT) and 4′- O -methyltransferase 2 (4′OMT2), which catalyse three methylation reactions to convert ( R,S )-norlaudanosoline to ( R,S )-reticuline. The committed step of BIA synthesis in plants is the condensation of the L -tyrosine derivatives L -dopamine and 4-hydroxyphenylacetaldehyde to produce ( S )-norcoclaurine, catalysed by the enzyme ( S )-norcoclaurine synthase ( Supplementary Fig. 1 ). The enzymatic synthesis of ( S )-norcoclaurine has not yet been achieved in S. cerevisiae , however, the 3′-hydroxylated analogue norlaudanosoline can be used to bypass synthesis of ( S )-norcoclaurine and the P450 NMCH, N- methylcoclaurine hydroxylase (CYP80B1), during pathway development [22] . The enzymes 6OMT, CNMT and 4′OMT2 from P. somniferum can be functionally co-expressed in yeast for the synthesis of racemic reticuline from ( R,S )-norlaudanosoline [22] . Strain GCY1086, expressing Block 1 enzymes from a plasmid, was incubated with ( R,S )-norlaudanosoline. The end product reticuline was produced with a yield of 20% ( Figs 3a and 4a ), twice the previously reported yield [22] . While Block 1 enzymes are predicted to function in plants in the order depicted in Supplementary Fig. 1 , a multitude of single- and double-methylated products can be formed when these enzymes are expressed in S. cerevisiae and incubated with norlaudanosoline [22] , [31] , [32] . For example, the three methyltransferases expressed in Block 1 can accept norlaudanosoline as a substrate and acceptance of N -methylnorlaudanosoline (laudanosoline) by both 6OMT and 4′OMT was also demonstrated [22] . We did not detect any single-methylated products ( m/z =302), and estimated the accumulation of double-methylated products ( m/z =316) to be 2%. Low accumulation of intermediates indicated that the limiting reaction of Block 1 is likely the first methylation event. This limitation could be due to the fact that norlaudanosoline is not a natural substrate or that intracellular norlaudanosoline is low due to poor transport. When wild-type cells were incubated with norlaudanosoline, 3% was initially found in the cell extract, which increased to just 10% after 16 h of incubation ( Supplementary Fig. 2A ), suggesting that substrate availability to the intracellular enzymes is low. 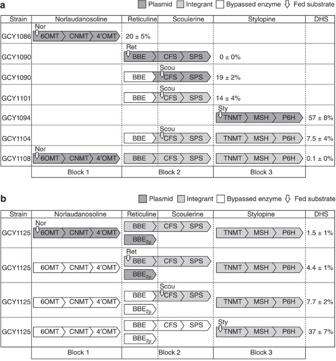Figure 3: BIA yields from engineered strains incubated with pathway intermediates. (a) BIA yields from cell-feeding assays of strains expressing Block 1, 2 and 3 individually or in combinations. (b) Cell-feeding assays of strain GCY1125 with one of the four different substrates, (R,S)-norlaudanosoline (nor), (S)-reticuline (ret), (S)-scoulerine (scou), (S)-stylopine (sty). Percent yield of end product is indicated in the appropriate column. Percent conversion was calculated as the ratio of total moles of end product recovered (sum of both cell extract and supernatant) to moles of supplemented substrate. Enzyme expressed from plasmid (dark grey); enzyme expressed from chromosome (light grey); enzymes expressed but not necessary for substrate conversion (no shading). BBE2μsignifies BBE expression from a 2μ vector. Data presented represent the mean±s.d. of at least three biological replicates. Figure 3: BIA yields from engineered strains incubated with pathway intermediates. ( a ) BIA yields from cell-feeding assays of strains expressing Block 1, 2 and 3 individually or in combinations. ( b ) Cell-feeding assays of strain GCY1125 with one of the four different substrates, ( R,S )-norlaudanosoline (nor), ( S )-reticuline (ret), ( S )-scoulerine (scou), ( S )-stylopine (sty). Percent yield of end product is indicated in the appropriate column. Percent conversion was calculated as the ratio of total moles of end product recovered (sum of both cell extract and supernatant) to moles of supplemented substrate. Enzyme expressed from plasmid (dark grey); enzyme expressed from chromosome (light grey); enzymes expressed but not necessary for substrate conversion (no shading). BBE 2μ signifies BBE expression from a 2μ vector. Data presented represent the mean±s.d. of at least three biological replicates. 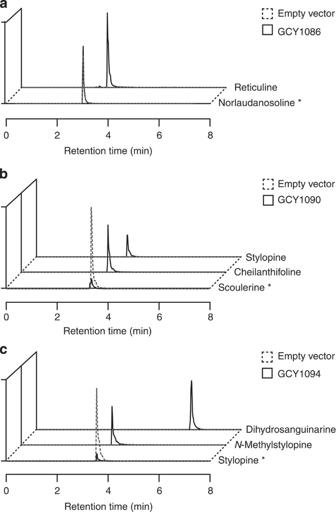Figure 4: LC-FT-MS profiles of BIAs from cell-feeding assays. (a) Cell-feeding assay of strain GCY1086 harbouring Block 1 enzymes and incubated with (R,S)-norlaudanosoline (*). (b) Cell-feeding assay of strain GCY1090 harbouring Block 2 enzymes and incubated with (S)-scoulerine (*). (c) Cell-feeding assay of strain GCY1094 harbouring Block 3 enzymes and incubated with (S)-stylopine (*). Chromatograms shown are the summed ion counts of supernatant and cell extract. Full size image Figure 4: LC-FT-MS profiles of BIAs from cell-feeding assays. ( a ) Cell-feeding assay of strain GCY1086 harbouring Block 1 enzymes and incubated with ( R,S )-norlaudanosoline (*). ( b ) Cell-feeding assay of strain GCY1090 harbouring Block 2 enzymes and incubated with ( S )-scoulerine (*). ( c ) Cell-feeding assay of strain GCY1094 harbouring Block 3 enzymes and incubated with ( S )-stylopine (*). Chromatograms shown are the summed ion counts of supernatant and cell extract. Full size image Block 2 contains the P. somniferum enzymes berberine bridge enzyme (BBE), CFS and SPS. In plants, the flavoprotein oxidase BBE stereoselectively converts ( S )-reticuline to ( S )-scoulerine [33] . A truncated version of BBE (PsBBEΔN) was cloned with CFS and SPSΔN into plasmid pGC994 ( Table 1 ). When cells expressing enzymes of Block 2 and CPR (strain GCY1090) were incubated with ( S )-reticuline, no scoulerine, cheilanthifoline or stylopine were detected ( Fig. 3a ), suggesting that initial conversion of ( S )-reticuline to scoulerine was poor. We hypothesized that BBEΔN activity was limiting the flux of Block 2. To assess the function of CFS and SPSΔN, we bypassed BBEΔN by feeding the next pathway intermediate, ( S )-scoulerine, to the same yeast strain. Here, we observed the accumulation of cheilanthifoline and 19% conversion of scoulerine to stylopine ( Figs 3a and 4b ), confirming that BBEΔN was limiting. We estimated 70% conversion to cheilanthifoline using a stylopine standard curve. Cheilanthifoline was mainly found in the supernatant while stylopine was predominantly found in the cell extract ( Supplementary Fig. 2B ). Accumulation of cheilanthifoline during cell-feeding assays also indicated that low activity of the SPS was limiting the flux of scoulerine to stylopine. The third block encodes the three enzymes catalysing the conversion of stylopine to dihydrosanguinarine. Stylopine is N -methylated to ( S )- cis - N -methylstylopine by TNMT [34] . The next two biosynthetic steps are catalysed by the P450 hydroxylases ( S )- cis - N -methylstylopine 14-hydroxylase (MSH) and protopine 6-hydroxylase (P6H). Both enzymes were recently identified and characterized from P. somniferum and Eschscholzia californica , respectively (CYP82N4 and CYP82N2v2) [25] , [27] . 6-Hydroxyprotopine spontaneously rearranges to dihydrosanguinarine. When cells expressing Block 3 and CPR (strain GCY1094) were incubated with ( S )-stylopine, the majority of the stylopine was consumed, resulting in 57% conversion to dihydrosanguinarine ( Figs 3a and 4c ). N -methylstylopine was the intermediate with the next largest peak area ( Fig. 4c ) and trace amounts of protopine were detected. We also detected 3% conversion to sanguinarine indicating spontaneous conversion of dihydrosanguinarine to sanguinarine. Approximately 55% of the pathway intermediate N -methylstylopine was found in the culture supernatant as opposed to stylopine and dihydrosanguinarine, which were mostly found in the cellular extract fraction ( Supplementary Fig. 2B ). This suggests that the charged intermediate N -methylstylopine is secreted outside of the cell, thereby reducing the pathway efficiency. Integration of Block 2 and Block 3 in the genome The vectors harbouring Blocks 1, 2, 3 and CPR are closely related and share several of the same promoters and terminators. We occasionally observed loss of function from strains harbouring multiple plasmids, which we attributed to recombination. To address this problem, Blocks 2 and 3 were integrated into the genome of S. cerevisiae ( Table 1 and Supplementary Table 1 ). Since the plasmids were single copy and the regions targeted for integration of the blocks had been demonstrated to allow for good expression [35] , we expected that the enzyme activity would not be affected by integration. Block 2 was integrated into S. cerevisiae and the strain was transformed with CPR (strain GCY1101). When incubated with scoulerine, 14% of the substrate was converted to stylopine, which is comparable to what was obtained by expressing Block 2 from a centromeric plasmid ( Fig. 3a ). Only trace cheilanthifoline and stylopine accumulation was observed in the absence of the heterologously expressed CPR, indicating the importance of including a cognate CPR for improved cytochrome P450 activity in S. cerevisiae. Block 3 was integrated into the Block 2 strain, generating a Block 2–Block 3 double integrant, which was subsequently transformed with CPR (strain GCY1104). Incubation of this strain with ( S )-scoulerine resulted in 7.5% conversion to dihydrosanguinarine ( Figs 3a and 5a ), which is an eight-fold decrease in dihydrosanguinarine synthesis compared with cells expressing Block 3 enzymes and incubated with ( S )-stylopine ( Fig. 3a ). Similar to previous feeding assays where cells expressed only Block 3 enzymes, the intermediate N -methylstylopine accumulated and trace protopine was detected ( Fig. 5a ). 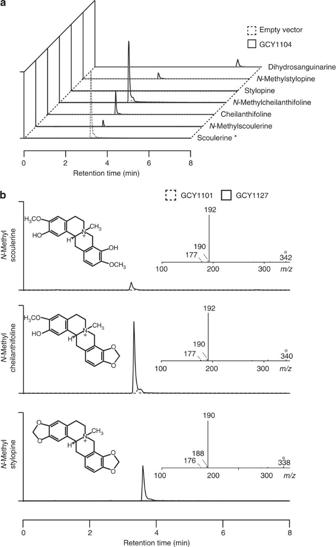Figure 5: LC-MS analysis of alkaloidsN-methylated by TNMT. (a) Cell-feeding assay of strain GCY1104 harbouring Block 2 and 3 enzymes and incubated with (S)-scoulerine (*) demonstrates the accumulation of the side-productsN-methylscoulerine andN-cheilanthifoline. (b) LC-FT-MS chromatographic profiles and fragmentation profiles of BIAs from cell-feeding assays of strains GCY1101 and GCY1127 incubated with (S)-scoulerine. In strain GCY1127 but not GCY1101, the productsN-methylscoulerine,N-methylcheilanthifoline andN-methylstylopine were detected. Chromatograms shown are the summed ion counts of supernatant and cell extract. Parent ion: · Figure 5: LC-MS analysis of alkaloids N -methylated by TNMT. ( a ) Cell-feeding assay of strain GCY1104 harbouring Block 2 and 3 enzymes and incubated with ( S )-scoulerine (*) demonstrates the accumulation of the side-products N -methylscoulerine and N -cheilanthifoline. ( b ) LC-FT-MS chromatographic profiles and fragmentation profiles of BIAs from cell-feeding assays of strains GCY1101 and GCY1127 incubated with ( S )-scoulerine. In strain GCY1127 but not GCY1101, the products N -methylscoulerine, N -methylcheilanthifoline and N -methylstylopine were detected. Chromatograms shown are the summed ion counts of supernatant and cell extract. Parent ion: · Full size image TNMT N -methylates scoulerine and cheilanthifoline When cells of the Block 2–Block 3 double integrant were incubated with ( S )-scoulerine, compounds with exact masses of 342.1710 m/z and 340.1548 m/z were detected in addition to expected sanguinarine pathway intermediates. These exact masses, and their fragmentation profiles, correspond to N -methylscoulerine and N -methylcheilanthifoline, respectively [36] . The compounds had been previously identified in opium poppy cell culture and were predicted to be a product of TNMT activity, an enzyme that had also been shown to methylate ( S )-canadine [34] . To confirm that TNMT was responsible for the N -methylation of cheilanthifoline and scoulerine, we compared the Block 2 integrant strain harbouring CPR on a plasmid (strain GCY1101) with the Block 2 integrant strain harbouring both CPR and TNMT on a plasmid (strain GCY1127). The resulting chromatograms and fragmentation profiles ( Fig. 5b ) for N -methylscoulerine, N -methylcheilanthifoline and N -methylstylopine demonstrate that all three compounds are present only in the presence of TNMT. These data provide the first experimental evidence that TNMT accepts both scoulerine and cheilanthifoline as substrates for methylation. Because we lacked standards to quantify the N -methylated products and since the three compounds are similar in structure, we assumed equal ionization efficiency and estimated their relative proportions by peak area: when strain GCY1127 is fed ( S )-scoulerine, the expected product N -methylstylopine is 33%, while N -methylscoulerine is 7% and N -methylcheilanthifoline is 60% ( Fig. 5b ). Diversion of the intermediates scoulerine and cheilanthifoline from dihydrosanguinarine synthesis affects the efficiency of the pathway and shows that favouring N -methylation of stylopine will be necessary to increase yield to the desired downstream compounds. Production of dihydrosanguinarine from norlaudanosoline The three functional blocks were combined to assemble a complete dihydrosanguinarine pathway in yeast. The Block 2–Block 3 integrant served as a background strain for the transformation of Block 1 and CPR (strain GCY1108). When this strain was incubated with ( R,S )-norlaudanosoline, trace levels of dihydrosanguinarine were observed ( Fig. 3a ), along with 13% conversion to reticuline and no other accumulation of downstream intermediates or N -methylated side products. Lack of conversion of endogenously synthesized ( R,S )-reticuline to scoulerine confirmed that BBEΔN was not highly active in our system, as previously observed by incubating cells expressing Block 2 enzymes with (S)-reticuline ( Fig. 3a ). In previous studies, BBEΔN has been functionally expressed from a high-copy vector [20] , [22] , which suggested that the expression level from a centromeric plasmid was insufficient for conversion of reticuline to scoulerine. To test this hypothesis, we co-transformed a high-copy vector expressing BBEΔN along with Block 1 and CPR plasmids into the double integrant (strain GCY1125). When strain GCY1125 was incubated with ( R,S )-norlaudanosoline, conversion to dihydrosanguinarine improved from trace to 1.5% ( Fig. 4a ) and ( R , S )-reticuline accumulation dropped from 13% to 0.5%, confirming that low BBEΔN expression was limiting flux. PsBBE was previously proposed to be functionally identical to E. californica BBE [26] , [37] , which is enantioselective for ( S )-reticuline [33] . However, more reticuline than expected was consumed assuming an equal mixture of ( R )- and ( S )-reticuline from ( R,S )-norlaudanosoline [22] , indicating that ( R )-reticuline is also consumed in our system. Finally, we independently incubated GCY1125 cells with ( R,S )-norlaudanosoline, ( S )-reticuline, ( S )-scoulerine or ( S )-stylopine to assess the efficiency of substrate conversion at different points in the complete pathway ( Fig. 3b ). In all GCY1125 substrate feeding experiments, spontaneous oxidation of dihydrosanguinarine to sanguinarine was detected, corresponding to 6% of the total dihydrosanguinarine. Feeding ( R,S )-norlaudanosoline resulted in 1.5% conversion to dihydrosanguinarine, while bypassing Block 1 using ( S )-reticuline resulted in 4% conversion to dihydrosanguinarine. Bypassing BBEΔN by incubating the same strain with ( S )-scoulerine increased conversion to only 8%. In all cases, the accumulation of the N -methylated side-products, especially N -methylcheilanthifoline, diverted intermediates from the dihydrosanguinarine pathway. In fact, the biggest increase in efficiency was observed when strain GCY1125 was incubated with stylopine, bypassing production of scoulerine and cheilanthifoline and their N -methylated products: from 8% to 35%. However, 35% yield is a decrease from the 57% yield observed when Block 3 enzymes were expressed on their own, indicating that expression of Block 1 and 2 negatively affects the yield of Block 3. Plant secondary metabolites are a rich source of bioactive molecules. The chemical diversity of these compounds derives from enzymes that have diversified to perform an array of stereo- and enantioselective modifications. Coupling these reactions by chemical synthesis to reach high yields can be difficult if not impossible. While plants remain the main source of these valuable natural compounds, the use of microbial platform has emerged as an attractive alternative. In this work, we described the reconstitution of a complex BIA biosynthetic pathway in S. cerevisiae . The sanguinarine pathway from norlaudanosoline includes four plant cytochrome P450s, enzymes that are difficult to functionally express in microbial systems [21] , [38] . While CFS, MSH and P6H were expressed in S. cerevisiae , the SPS enzyme required substitution of the N-terminal membrane-spanning domain in order to achieve sufficient expression. However, SPS remained a limiting enzyme in Block 2, resulting in a build-up of cheilanthifoline, which was diverted to N -methylcheilanthifoline in the presence of TNMT. Increasing the activity of SPS, and thus the flux of alkaloids towards sanguinarine, is a key point of optimization in this pathway. Orthologous genes from different plants can have varying kinetic constants and expression efficiency in yeast. Searching transcriptomics databases for orthologous SPS candidates [28] , [39] may provide a good option for optimizing pathway efficiency and flux to the desired end-product. Moreover, cytochrome b 5 has been reported to enhance activity of certain cytochrome P450s (ref. 40 ). Tuning expression of the four P450s, CPR and cognate cytochrome b 5 could increase pathway efficiency. The high number of P450s expressed in this work may be affecting yields of dihydrosanguinarine. ( S )-Scoulerine fed to Block 2–Block 3 integrant strains expressing four P450s yielded the same conversion to dihydrosanguinarine whether or not Block 1 and BBEΔN-2μ were expressed (7.5 vs 7.7%; Fig. 3 ). In contrast, conversion of the fed substrate ( S )-stylopine to dihydrosanguinarine dropped from 57% when Block 3 enzymes were expressed in isolation to 37% when Block 3 enzymes were co-expressed with Block 1, BBEΔN-2μ and integrated Block 2. Because Block 1 and BBEΔN-2μ do not appear to affect yields, we hypothesize that it was the co-expression of Block 2 with Block 3 that was responsible for this decrease in yields. Further, because these two strains were fed stylopine, the promiscuity of TNMT is not responsible for this decrease. This suggests that it is the co-expression of the four P450s in Blocks 2 and 3 in GCY1125 that is decreasing pathway efficiency. Synthesis of the side products N -methylcheilanthifoline and N -methylscoulerine by TNMT was shown to be a major limiting factor in the reconstituted pathway. Promiscuity is a common theme among enzymes involved in plant-specialized metabolism and is one of the factors contributing to the great chemodiversity of plant secondary metabolites [41] . While broad substrate specificity of PsTNMT had been previously described [34] , we present the first experimental evidence of its acceptance of scoulerine and cheilanthifoline as substrates. Possible solutions for overcoming the problem of PsTNMT promiscuity in our system would include screening for orthologous plant enzymes with narrower substrate specificity, enzyme engineering [42] , substrate channelling and/or spatio-temporal sequestration of the reactions [43] , [44] . While N -methylscoulerine and N -methylcheilanthifoline are undesirable side-products, they may themselves be end products of interest. Both compounds are quaternary BIAs like sanguinarine and berberine. N -methylscoulerine (cyclanoline) can be extracted from several plants of the genus Stephania and has been described as an acetylcholinesterase inhibitor [45] , but to the best of our knowledge N -methylcheilanthifoline has never been detected in plants. The promiscuity of TNMT could also be further explored to generate other quarternary BIAs. Synthesis of N -methylcheilanthifoline, although serendipitous, highlights the potential of combinatorial biology in S. cerevisiae , through which libraries of alkaloids can be generated independent of their abundance in nature. Synthesis of ( S )-reticuline from glucose and glycerol has been reported in E. coli [18] , [19] but not in S. cerevisiae . Thus, supplemented ( R,S )-norlaudanosoline was required to measure the efficiency of the reconstituted BIA pathway. We observed that just 10% of fed norlaudanosoline was detected in the cell extract after 16 h of incubation with the negative control yeast cells ( Supplementary Fig. 2A ). While we cannot directly compare substrates with different chemical properties and possibly different mechanisms of transport into yeast, we suspect that limited availability of norlaudanosoline to the intracellular enzymes is limiting pathway efficiency. In a previous study, it was shown that ( R,S )-reticuline accumulation increased with ( R,S )-norlaudanosoline concentration in cell-feeding assays [22] , further supporting the evidence that low intracellular norlaudanosoline concentration is limiting flux. Linking the reconstituted alkaloid pathway to the microbe’s central metabolism, thereby bypassing the need to feed norlaudanosoline, will likely boost yields of reticuline and thus the entire dihydrosanguinarine pathway. Next-generation sequencing technology and the accelerated discovery of genes combined with advances in synthetic biology is opening up new opportunities for the reconstitution of plant natural product biosynthetic pathways in microbes [46] . In the last 5 years, there has been a growing trend in the complexity and diversity of the chemical structures achieved by these pathways. For example, microbes have been engineered for the synthesis of terpenoids such as artemisinin acid [10] and taxa-di-ene [47] , BIAs such as magnoflorine [20] and canadine [22] and glucosinates such as indolylglucosinolate [48] . Cytochrome P450s are required for the synthesis of a wide range of plant natural products and the efficient recombinant expression of this class of enzyme can be difficult. Of all pathways reconstituted in microbes thus far, only those of the mammalian hydrocortisone [49] and plant dihydrosanguinarine pathways require the heterologous expression of four cytochrome P450s. The dihydrosanguinarine pathway described in this work represents the most complex plant alkaloid biosynthetic pathway ever reconstituted in yeast and provides a glimpse into the potential of engineering microbes for the synthesis of ever more complex plant natural products. Chemicals and reagents ( S )-Reticuline was a gift from Johnson & Johnson. ( R,S )-Norlaudanosoline was purchased from Enamine Ltd. (Kiev, Ukraine), ( S )-scoulerine and ( S )-stylopine from ChromaDex (Irvine, CA, USA), protopine from TRC Inc. (North York, Ontario, Canada) and sanguinarine from Sigma. Dihydrosanguinarine was prepared by NaBH 4 reduction of sanguinarine [50] . Antibiotics, growth media and α- D -glucose were purchased from Sigma-Aldrich. Restriction enzymes, T4 DNA polymerase and T4 DNA ligase were from New England Biolabs (NEB). Polymerase chain reactions (PCRs) for the assembly of expression cassettes were performed using Phusion High-Fidelity DNA polymerase (NEB/Thermo Scientific). Taq polymerase (Fermentas/Thermo Scientific) was used in PCRs confirming DNA assembly or chromosomal integration. PCR-amplified products were gel purified using the QIAquick purification kit (Qiagen). Plasmid extractions were done using the GeneJET plasmid mini-prep kit (Thermo Scientific). Genomic DNA preparations were done using the DNeasy blood and tissue kit (Qiagen). HPLC-grade water was purchased from Fluka. HPLC-grade methanol and acetonitrile were purchased from Fischer Scientific. Identification and characterization of PsCFS and PsSPS RNA extraction from root or stems of the P. somniferum (opium poppy) cultivar Bea’s Choice was performed using a modified CTAB method [51] and the cDNA libraries were constructed using the TruSeq Stranded mRNA Sample Prep Kit (Illumina). Illumina GA sequencing was performed with 7 pmol per library with one lane in the flow cell. Sequence trimming was done with Cutadapt [52] and assembled with Velvet-Oases v0.1.16 (ref. 53) [53] and the clustering tools CD-HIT-EST [54] and CAP3 (ref. 55) [55] . Gene expression analysis was performed by re-mapping the raw reads to the assembled contigs using Bowtie [56] and further refined using the RNA-seq by Expectation–Maximization package [57] . The pESC-CPR vector encoding opium poppy cytochrome P450 reductase (PsCPR) fused to a c-Myc tag was used for the heterologous expression of plant proteins in S. cerevisiae [25] . PsCFS ( CYP719A25 ; GenBank ADB89213) was amplified from opium poppy cell culture cDNA using the primer listed in Supplementary Table 3 . The amplicon was inserted into Not I and Spe I restriction sites of pESC-CPR in-frame with a FLAG-tag sequence yielding pESC-CPR/CFS. A synthetic PsSPS ( CYP719A20 ) gene (GenBank KF481962), codon-optimized for expression in S. cerevisiae and containing a sequence encoding the N-terminal membrane-spanning domain from the Lactuca sativa (lettuce) germacrene A oxidase (43 amino acids) [58] replacing the corresponding native domain (29 amino acids) to increase protein stability [59] , was inserted into the Not I and Spe I restriction sites of pESC-CPR [25] in-frame with a FLAG-tag sequence yielding pESC-CPR/SPSΔN. For heterologous gene expression, S. cerevisiae strain YPH499, harbouring the plasmid of interest, was grown in yeast nitrogen broth, synthetic dropout supplement lacking leucine, 0.2% D -glucose, 1.8% D -galactose and 1% D -raffinose for 48 h at 30 °C [25] . Microsomes were prepared by glass bead disruption and ultracentrifugation [38] . Cytochrome P450 enzyme assays were performed with 20 μg of microsomal protein in 50 mM HEPES, pH 7.5, 125 μM ( S )-scoulerine and 500 μM NADPH in 50 μl at 30 °C. Reactions were stopped after 90 min with the addition of 100 μl MeOH and the precipitate was discarded. The supernatant was evaporated to dryness and suspended in 50 μl solvent A (95:5, 10 mM ammonium acetate, pH 5.5:acetonitrile). Reconstitution of the sanguinarine pathway in S. cerevisiae For liquid cultures, S. cerevisiae was grown in yeast nitrogen broth, synthetic dropout supplement, 2% α- D -glucose and amino acids as appropriate (YNB-DO-GLU) at 30 °C and 200 r.p.m. For solid media, selection for plasmid transformation was on YNB-DO-GLU/agar, while selection for chromosomal integration was on YPD/agar (yeast extract peptone-dextrose) with the appropriate antibiotic. Transformations were either performed by heat shock in the presence of lithium acetate, carrier DNA and PEG 3350 (ref. 60) [60] , or by electroporation in the presence of sorbitol [9] . All coding sequences are from P. somniferum with the exception of P6H, which is from E. californica . Synthetic sequences of Ps6OMT (GenBank KF554144), Ps4 ′ OMT2 (GenBank KF661327), PsCNMT (GenBank KF661326) and PsP450R(CPR) (GenBank KF661328) were codon-optimized by DNA2.0 for optimal expression in yeast. The lettuce germacrene A oxidase N-terminus membrane-spanning domain was incorporated into SPS as described above and 25 amino acids were truncated from N-terminus of the opium poppy BBE ( PsBBE Δ N ) [22] , [61] . When not otherwise specified, coding sequences in Table 1 and Supplementary Table 1 correspond to the plant cDNA sequences. The partial Kozak sequence AAAACA was introduced upstream of all coding sequences by PCR or as an integral part of gene synthesis. Assembly of plasmids by homologous recombination Blocks of enzymes were designed to independently express sequential enzymes of the dihydrosanguinarine pathway. Enzyme blocks were cloned into the pGREG series of E. coli – S. cerevisiae shuttle vectors [62] . Vectors pGREG503, 504, 505 and 506, harbouring the HIS3 , TRP1 , LEU2 and URA3 auxotrophic markers, respectively, were modified by site-directed mutagenesis to contain a unique Kpn I site at the 3′ end of a stuffer cassette in the multiple cloning site using the PCR primers reported in Supplementary Table 2 . Gene expression cassettes were inserted by homologous recombination into pGREG vectors previously linearized with Asc I/ Kpn I. Empty pGREG control plasmids were created by intra-molecular ligation of the linearized pGREG made blunt with T4 DNA polymerase. The DNA assembler technique, which takes advantage of in vivo homologous recombination in yeast [9] , was used for the assembly of the sanguinarine pathway. Promoters, genes and terminators were assembled by incorporating a ~50-bp homologous region between the segments. Expression cassettes were joined to each other and to the vector backbone using DNA linkers (C6-H(n)-C1 linkers in Supplementary Table 3 ), with the exception of some components of Block 3. DNA linkers were added to promoters and terminators by PCR using the primers listed in Supplementary Table 3 and CEN.PK genomic DNA as template. In addition, a Not I site was introduced in the 3′ linker primer containing homology to pGREG backbones, allowing the excision of enzyme blocks by Asc I/ Not I double digest. PsBBE Δ N was also independently cloned into the 2μ high copy vector pYES2. For DNA assembly, the pYES2 backbone was amplified by PCR using primers pYES2 for and pYES2 rev described in Supplementary Table 3 . Transformation of DNA fragments in yeast for homologous recombination was accomplished by electroporation. Assembled plasmids were transferred to E. coli and sequenced-verified. All the plasmids used in this work are described in Table 1 and Supplementary Table 1 . Integration of enzyme blocks into the genome Integration of enzyme blocks into the genome of S. cerevisiae was achieved through targeted homologous recombination to integration sites shown to support relatively high levels of gene expression [35] . Enzyme blocks were integrated into the genome using upstream and downstream homology regions, selection cassettes and gene cassettes, as parts for chromosomal DNA assembly [9] . Selection cassettes Hyg R and G418 R (for Blocks 2 and 3, respectively), were amplified from pZC3 and pUG6, while genomic homology regions (site 18 on chromosome XV and site 20 on chromosome XVI for Blocks 2 and 3, respectively) were amplified from CEN.PK genomic DNA using primers described in Supplementary Table 4 . Gene cassettes of Blocks 2 and 3 were excised from their plasmids by Asc I// Not I-HF/ Xba I digestion. Parts for assembly were transformed into S. cerevisiae by the lithium acetate method and integrants were selected on solid media. Successful integration was verified by PCR using genomic DNA as template. Cell-feeding assays Whole-cell substrate feeding assays were used to test the function of each enzyme block individually and in combinations. To prepare the cells for the feeding assays, a colony of S. cerevisiae was inoculated in YNB-DO-GLU and incubated for 24 h. Cultures were diluted to an OD 600 of 0.8 into 6 ml of fresh YNB-DO-GLU and incubated for an additional 7 h. Cells were harvested by centrifugation at 2,000 g for 2 min. Supernatants were decanted and cells were suspended in 2 ml of Tris-EDTA (10 mM Tris–HCl, 1 mM EDTA, pH 8), containing 10 μM of one of the following feeding substrates: ( R,S )-norlaudanosoline, ( S )-reticuline, ( S )-scoulerine or ( S )-stylopine. Cells were incubated for 16 h then harvested by centrifugation at 15,000 g for 1 min. For BIA extraction from cells, the cell pellet was suspended in 500 μl methanol with ~50 μl acid-washed glass beads and vortexed for 30 min. Cell extracts were clarified by centrifugation at 15,000 g for 1 min and used directly for LC-MS analysis. MRM analysis of alkaloids Analysis of enzyme assays was performed using an Agilent 1200 liquid chromatography system equipped with a 6410 triple-quadrupole mass spectrometer (Agilent Technologies, Santa Clara, CA). Solvent A1 (95:5, 10 mM ammonium acetate, pH5.5:acetonitrile) and solvent B (100% acetonitrile) were used in a gradient elution to separate the metabolites of interest as follows: 0–6 min at 0–60% B (linear gradient), 6–7 min at 99% B, 8–8.1 min at 100% A1, followed by a 3.9 min equilibration at 100% A1. Ten microlitres of either cell extract or supernatant fraction were loaded on the HPLC column run at a flow rate of 0.7 ml min −1 . Following liquid chromatography (LC) separation, the eluate was applied to the mass analyser using the following parameters: capillary voltage, 4,000 V; fragmentor voltage, 125 V; source temperature, 350 °C; nebulizer pressure, 50 psi; gas flow, 10 l min −1 . Scoulerine, cheilanthifoline and stylopine were detected in MRM (multiple reaction monitoring) mode using a collision energy of 25 eV and monitored transitions of m/z 328→178, 326→178 and 324→176, respectively. FT-MS analysis of alkaloids Detection of alkaloids in the sanguinarine biosynthetic pathway was performed by FT-MS using a 7T-LTQ FT ICR instrument (Thermo Scientific, Bremen, Germany). Alkaloids were separated by reverse-phase HPLC (Perkin Elmer SERIES 200 Micropump, Perkin Elmer, Norfolk, CT, USA) using an Agilent Zorbax Rapid Resolution HT C18 2.1*30 mm, 1.8 micron column. Solvent A2 (0.1% acetic acid) and solvent B (100% acetonitrile) were used in a gradient elution to separate the metabolites of interest as follows: 0–1 min at 100% A2, 1–6 min at 0–95% B (linear gradient), 7–8 min at 95% B, 8–8.2 min at 100% A2, followed by a 1 min equilibration at 100% A2. Three microlitres of either cell extract or supernatant fraction was loaded on the HPLC column run at a flow rate of 0.25 ml min −1 . Dilutions in methanol were performed to keep alkaloid concentrations within the range of standard curve values and avoid saturating FT signals. Following LC separation, metabolites were injected into the LTQ-FT-MS (ESI source in positive ion mode) using the following parameters: resolution, 100,000; scanning range, 250–450 AMU; capillary voltage, 5 kV; source temperature, 350 °C; AGC target setting for full MS were set at 5 × 10 5 ions. Identification of alkaloids was done using retention time and exact mass (<2 p.p.m.) of the monoisotopic mass of the protonated molecular ion [M + H] + . LC-FT-MS data were processed using the freely available program Maven [63] . When available authentic standards were used to confirm the identity of the BIA intermediates (using HPLC retention times and exact masses) and to quantify sanguinarine alkaloids. When unavailable, we assumed equal ionization efficiency between an intermediate and the closest available quantifiable alkaloid ( m/z 302 and m/z =316 as reticuline; cheilanthifoline as stylopine). How to cite this article: Fossati, E. et al. Reconstitution of a 10-gene pathway for synthesis of the plant alkaloid dihydrosanguinarine in Saccharomyces cerevisiae. Nat. Commun. 5:3283 doi: 10.1038/ncomms4283 (2014).